Topological structure dynamics revealing collective evolution in active nematics Topological defects frequently emerge in active matter like bacterial colonies, cytoskeleton extracts on substrates, self-propelled granular or colloidal layers and so on, but their dynamical properties and the relations to large-scale organization and fluctuations in these active systems are seldom touched. Here we reveal, through a simple model for active nematics using self-driven hard elliptic rods, that the excitation, annihilation and transportation of topological defects differ markedly from those in non-active media. These dynamical processes exhibit strong irreversibility in active nematics in the absence of detailed balance. Moreover, topological defects are the key factors in organizing large-scale dynamic structures and collective flows, resulting in multi-spatial temporal effects. These findings allow us to control the self-organization of active matter through topological structures. Topological defects are singular points or lines surrounded by spatially varying order parameter fields. They emerge as a local manifestation of spatial heterogeneity of large-scale order and play a critical role in determining the physical property of matters ranging from early universe to materials in our daily life [1] , [2] , [3] , [4] . Recently, they have also been widely observed in active matter composed of self-propelled entities in states of exotic collective motion [5] , [6] , [7] , [8] , [9] , [10] , [11] , [12] , [13] , [14] , [15] , [16] . Active matter represents a new state of matter where large-scale mass flow emerges through the self-organization of interacting self-propelled particles. One common feature in active systems is the abnormal large density fluctuations, which are accompanied with highly dynamical collective swirling and swarming motions of active particles [15] , [16] . The nematic state of active matter is of particular interest, where genuine giant number fluctuations are predicted by theory and verified in experiment on driven rods [10] , [17] . In the experiment by V. Narayan et al. [10] , the ballistic motion of topological defects is first observed and such motion shows the evidence of curvature-driven flows, which are predicted to be ubiquitous in active nematics [13] , [14] , [17] . In cytoskeleton mixtures, nematic aligned extensile microtubule bundles may spontaneously buckle, accompanied with the unbinding of topological defects [8] . It is well-known that, in equilibrium 2-dimensional (2D) system, the spontaneous unbinding of topological defects is a sign that the system enters into isotropic state [18] . In contrast to the well-known physical property of topological defects in equilibrium, in active system we still lack a clear picture of the route from the microscopic dynamics of active particles to their collective evolutions. Especially, despite knowledge about the collective motion of active nematics, it is still unclear how topological defects emerge and affect the exotic non-equilibrium behaviour in active nematics. Here, to explore the general behaviour of topological defects, we combine simulation and analytical methods to study a 2D system of self-driven granular elliptic rods on a substrate, where we take the effect of collisions among particles explicitly into account. The model is a particle-based dry active nematic system without media fluids. It eliminates the effects of fluid dynamics on particles, which facilitates the construction of a corresponding kinetic theory. We reveal not only general dynamics of topological structures but also their roles in large-scale collective motions in such active media. First, the self-driven motion, dissipation and mutual collisions among particles break detailed balance in active media. Without detailed balance, in the process of spontaneous creation of topological defect pair, local polar disclination hinders immediate reversible annihilation and triggers active unbinding of topological defect pair. Collective motion arises in response to asymmetrical ordered structures near topological defects, which also drive super-diffusive motion of polar defects. Second, we find that the time regime for large-scale relaxation coincides with the regime of super-diffusivity of polar disclination. The system is in a state of chaos with the emergence of large-scale particle flows driven by non-static curved nematic field whose dynamics is governed by the spontaneous excitation, transportation and annihilation of topological defects. Once they are spontaneously unbound, topological defects cannot be eliminated by local adjustment except through mutual annihilation of opposite disclinations. As a result, the dynamics of these topological structures likely govern the system’s giant number fluctuations and their relaxations. The close correspondence between the dynamics of topological defects and multi-spatial temporal effects of the relaxation suggests a way to control collective motion in active media through tracking and manipulating topological defects in real time. Excitation of topological defects in active nematics In 2D simulations of active nematics, we drive, typically, several thousands of hard elliptic rods along their own major axes. The driving force represents a simplification for the micro-driving along agitated rod or dragged filament [7] , [10] . To ensure head-tail symmetry of every particle, it can switch between forward and backward directions randomly after τ simulation sweeps on average (see Methods). In active nematic state, our simulations also observe typical topological defects shown in Fig. 1a–d . 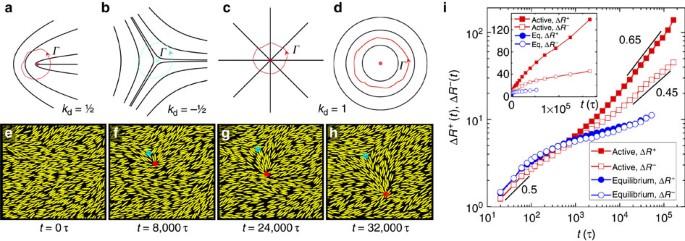Figure 1: Spontaneous excitation of topological defects and their dynamics. (a–d) Typical order parameter fields near the singular points of topological defects in 2D nematic state. If we follow a loop enclosing the singular point, we shall experience a total change of order parameter’s angleθbyds=2πkd, wheresis the distance on the loop Γ and the disclination numberkdindicates the strength of topological defect4. We have disclination number (a)kd=1/2, (b)kd=−1/2, (c)kd=1 (aster), and (d)kd=1 (vortex), respectively. (e–h) The process of the creation and separation of topological defects pair of disclinationkd=1/2 (red spot) and −1/2 (cyan spot) for the mean particle number densityρ=4.6. The polar disclinationkd=1/2 shows directional motion, while disclinationkd=−1/2 is relatively idle in moving as required by local symmetry. (i) Average motion of topological defects in log-log plot and linear plot (inset). In active media, disclinationskd=1/2 (red solid square) show superdiffusivity in long-time regime, whilekd=−1/2 (red square) exhibits weak subdiffusivity. Bothkd=1/2 and −1/2 in equilibrium show sub-diffusivity. Figure 1e-h displays a process of the spontaneous excitation of topological defect pairs k d =1/2 and − 1/2, which is created together obeying topological constraint in a formerly defect-free region. In the early stage ( Fig. 1f ), they are close to each other and distort the order-parameter field locally. Figure 1: Spontaneous excitation of topological defects and their dynamics. ( a – d ) Typical order parameter fields near the singular points of topological defects in 2D nematic state. If we follow a loop enclosing the singular point, we shall experience a total change of order parameter’s angle θ by d s =2π k d , where s is the distance on the loop Γ and the disclination number k d indicates the strength of topological defect [4] . We have disclination number ( a ) k d =1/2, ( b ) k d =−1/2, ( c ) k d =1 (aster), and ( d ) k d =1 (vortex), respectively. ( e – h ) The process of the creation and separation of topological defects pair of disclination k d =1/2 (red spot) and −1/2 (cyan spot) for the mean particle number density ρ =4.6. The polar disclination k d =1/2 shows directional motion, while disclination k d =−1/2 is relatively idle in moving as required by local symmetry. ( i ) Average motion of topological defects in log-log plot and linear plot (inset). In active media, disclinations k d =1/2 (red solid square) show superdiffusivity in long-time regime, while k d =−1/2 (red square) exhibits weak subdiffusivity. Both k d =1/2 and −1/2 in equilibrium show sub-diffusivity. Full size image Anomalous dynamics of topological defects In equilibrium 2D nematic state, emerging defect pair must be tightly bound and would be reversibly annihilated [18] , [19] . In active nematics, however, we observe a fast separation of topological defects created as a pair (see Fig. 1f–h ). To further qualitatively characterize the dynamic disparities between active and non-active media, we track the motions of topological defects in both systems (see Methods). Let us define as the average distance travelled by +1/2 and − 1/2 disclinations for a period t after their creation at time , respectively. and are the initial positions of +1/2 and −1/2 disclinations of the spontaneously created defect pair i , and disclinations’ lifetimes are and , respectively. if , else . In Fig. 1i , after an initial weak diffusive regime, we witness the supper-diffusive behaviour of +1/2 disclination, while −1/2 disclination exhibits weak subdiffusive behaviour in active media. In contrast, in non-active system, +1/2 disclination exhibits the same subdiffusive dynamics as −1/2 disclination. Thus, although topological defects in active system share the same mathematical description with their counterparts in non-active system, these same structures will give rise to totally different dynamical behaviours. Effects of micro-driving on the motion of defects To understand this major difference, let us focus on the microscopic level. We notice that in active media the presence of persistent micro-driving along a particle’s long axis breaks the detailed balance condition. As a result asymmetric structures may induce particle flows that are forbidden in equilibrium [10] , [20] , [21] , [22] . Here the asymmetric structures are self-emergent in the nematic field with the excitation of topological defect pairs. Defect of k d =1/2 with local polarity thus tends to move almost unidirectionally away from defect of k d =−1/2 after their co-emergence. In Fig. 2a–h , we measure how the kinetics of micro-driving affects the motion of defects. We start from a configuration with only a pair of defects (see Fig. 2e ) and track their motion. In Fig. 2a–d , the moving trajectories of defects convince the disparities between the dynamics of k d =−1/2 ( Fig. 2a,c ) and k d =+1/2 ( Fig. 2b,d ), as also demonstrated in Figure 1i . Further, with the increase of average driving velocity v 0 and persistent driving time τ , the motion of defect k d =1/2 speeds up significantly. As shown in Fig. 2g , the end-to-end distance Δ L for k d =1/2 grows with the increase of v 0 and τ . 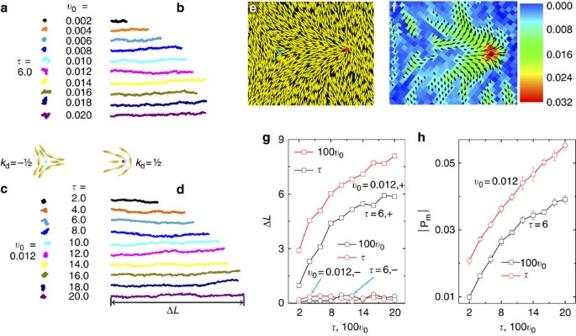Figure 2: The motion of a single pair of topological defects. (a–d) Moving trajectories of topological defects. (a) (kd=−1/2) and (b) (kd=1/2) are the trajectories for a fixedτ(=6.0) andv0varying from 0.002 to 0.02. (c) (kd=−1/2) and (d) (kd=1/2) are the cases whereτvaries from 2 to 20 withv0=0.012. All the simulations start from the same configuration as shown in (e), and run 2 × 105simulation sweeps. Every trajectory is obtained by averaging 10 independent runs. (e) Configuration of topological defects pair at the beginning of simulations. (f) Polarity field near topological defects. To obtain the polarity field in simulation, the system is coarse-grained into 60 × 60 periodic square lattice cells, each with side length 0.5 in particle length. The polarity field is obtained by averaging(which represents instantaneous driving direction of particle, see Methods) of particles whose centre of mass locate in local unit cell. The average is performed over 5 × 103(≫τ) continuous simulation sweeps and 100 independent runs starting from (e). Arrows indicate polar field in local unit cells. Both the colour scale and length of arrow indicate the magnitude of local polarity. (g) End-to-end distances ΔLof the moving trajectories of topological defects. (h) The maximum local polaritynear +1/2 defect extracted from the polar field as shown in (f). Figure 2: The motion of a single pair of topological defects. ( a – d ) Moving trajectories of topological defects. ( a ) ( k d =−1/2) and ( b ) ( k d =1/2) are the trajectories for a fixed τ (=6.0) and v 0 varying from 0.002 to 0.02. ( c ) ( k d =−1/2) and ( d ) ( k d =1/2) are the cases where τ varies from 2 to 20 with v 0 =0.012. All the simulations start from the same configuration as shown in ( e ), and run 2 × 10 5 simulation sweeps. Every trajectory is obtained by averaging 10 independent runs. ( e ) Configuration of topological defects pair at the beginning of simulations. ( f ) Polarity field near topological defects. To obtain the polarity field in simulation, the system is coarse-grained into 60 × 60 periodic square lattice cells, each with side length 0.5 in particle length. The polarity field is obtained by averaging (which represents instantaneous driving direction of particle, see Methods) of particles whose centre of mass locate in local unit cell. The average is performed over 5 × 10 3 ( ≫ τ) continuous simulation sweeps and 100 independent runs starting from ( e ). Arrows indicate polar field in local unit cells. Both the colour scale and length of arrow indicate the magnitude of local polarity. ( g ) End-to-end distances Δ L of the moving trajectories of topological defects. ( h ) The maximum local polarity near +1/2 defect extracted from the polar field as shown in ( f ). Full size image To elucidate the structural basis for the anomalous dynamics of topological defects, we calculate the distribution of local polarity field p ( r ) by coarse-graining and short-time averaging the simulation system. Figure 2f shows the snapshot of the polarity field p ( r ) near topological defect pair, where the maximum of p ( r ) locates near the discontinuity of defect k d =+1/2. For a finite τ , a simple analysis of Equation (7) shows that the distorted nematic alignment will induce the emergence of local polarity, which depends linearly on v 0 and τ (see supplementary Equation (15) in Supplementary Discussion ). In Fig. 2h , with the increase of τ and v 0 , we show the monotonic increase of maximum local polarity . Corresponding to the growth of Δ L as shown in Fig. 2g , such behaviour manifests that the weak but statistically significant polar arrangement of particles near k d =+1/2 defect favours to push the +1/2 defect away from −1/2 defect. The interaction and annihilation of topological defects With the excitation and active separation of disclinations, the interaction between disclinations and their mutual annihilations are unavoidable [23] , [24] (see Supplementary Movie 1 ). In Fig. 3a–c , we show typical snapshots for the collision process between polar disclinations and the formation of transient aster-like structure with disclination number k d =1. After that, in Fig. 3d , the aster degrades into two polar disclinations again. In Fig. 3e,f , annihilation of k d =1/2 and −1/2 takes place, resulting in remarkable transformation of local nematic director field. 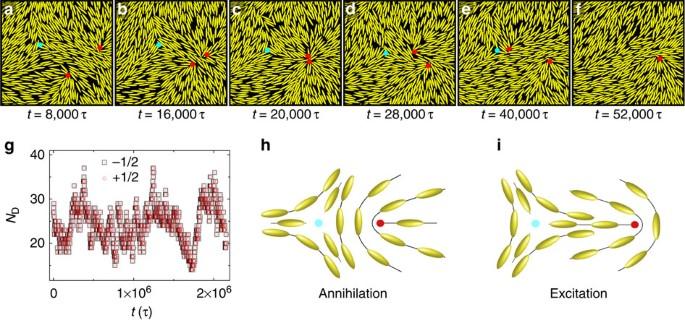Figure 3: Interaction and annihilation of topological defects. (a–c) Collision between two disclinations ofkd=1/2 and the formation of a transient aster (kd=1). (d–f) Decomposition of aster and annihilation ofkd=1/2 and−1/2. (g) Simulation time sequences of number of defects (ND) in the system forρ=4.6 in active simulation.kd=1/2 (red) and−1/2 (black) have the same number in the system. (h,i) Configurations of local particle arrangement, (h) before annihilation and (i) after excitation. Figure 3g shows the number of defects with significant fluctuations, revealing dynamical equilibrium between excitation and annihilation of disclinations. Figure 3: Interaction and annihilation of topological defects. ( a – c ) Collision between two disclinations of k d =1/2 and the formation of a transient aster ( k d =1). ( d – f ) Decomposition of aster and annihilation of k d =1/2 and − 1/2. ( g ) Simulation time sequences of number of defects ( N D ) in the system for ρ =4.6 in active simulation. k d =1/2 (red) and − 1/2 (black) have the same number in the system. ( h , i ) Configurations of local particle arrangement, ( h ) before annihilation and ( i ) after excitation. Full size image The annihilation process of disclination pair is not a simple reversion of its creation in such active media. Dynamical irreversibility will hinder the immediate annihilation of disclination pairs generated together. We notice that the configuration of disclination pair before its annihilation is different from that after its creation, as shown in Fig. 3e and Fig. 1f , respectively, which are also illustrated in Fig. 3h,i for clarity. After the spontaneous creation, the polar defect k d =1/2 is always on one of the apolar defect’s three branches (as shown in Fig. 3i ) and tends to move away from k d =−1/2. In the annihilation configuration (as shown in Fig. 3h ), the polar defect approaches the −1/2 defect through the valley between the latter’s two branches. Dynamically, these configurations greatly facilitate the corresponding processes. Instability and the microscopic collision processes A direct consequence of the spontaneous excitation of topological defect pairs and their irreversible separations is the breakdown of quasi-long-range nematic order. In Fig. 4a,b with the increase of mean particle number density ρ , we find that the order properties of active nematics are directly related to the quantities of topological defects. The measured appearant nematic order parameter is defined as the positive eigenvalue of matrix and nematic spatial correlation , where N is total particle number, u α ( i ) is the αth component of the i th particle orientation vector u ( i )=(cosθ i , sinθ i ) and r i is the position of its centre of mass. represent temporal average. As shown in Fig. 4a,b , to our surprise, we observe the breakdown of quasi-long-range nematic order in high density regime; in low density regime, however, the system achieves such order as indicated by the well-known power law decay, that is, g 2 ( r ) r − η . The non-active system, on the contrary, shows opposite tendency and attains topological order in high density regime. In accordance with the behaviours of and g 2 ( r ), we identify that the mean topological defect number increases with the breakdown of quasi-long-range order in active simulations (see the inset of Fig. 4a and snapshots of Fig. 4c,d ). 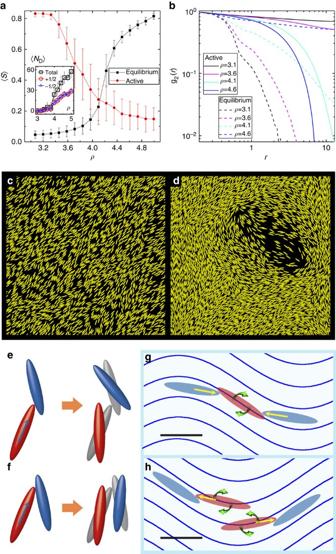Figure 4: Breakdown of topological nematic order in high density regime. (a) Transition curves offor active nematics (red) and equilibrium ones (black). The inset shows the mean number of topological defects in active simulations, where mean total number (black) is the sum of the numbers forkd=1/2 (red) andkd=−1/2 (blue). (b)g2(r) for active (solid curve) and equilibrium (dashed curve) systems. Active system only exhibits algebraic order in low density regime. (c,d) Simulation snapshots for active system with (c)ρ=3.1 and (d)ρ=4.6. Note the transient excitation of vortex ind. (e,f) Driving-induced collision processes in highly dissipative system. The blue arrows indicate the direction of motion for particles on collision. Grey particles indicate the configurations before collision. Particle rotations depend on relative positions and angles between particles. Ine, the colliding particle (red) tends to align with the collided particle (blue), while the collided particle tends to rotate away. Inf, both particles align with each other. (g,h) Two different processes causing the instability of nematic alignment. Black lines indicate the bulk nematic alignment. Blue curves indicate the bending deformations of nematic alignment caused by fluctuations. Yellow arrows indicate the direction of motion for particles on collision. Green arrows indicate the direction of particle’s rotation caused by collision. Figure 4: Breakdown of topological nematic order in high density regime. ( a ) Transition curves of for active nematics (red) and equilibrium ones (black). The inset shows the mean number of topological defects in active simulations, where mean total number (black) is the sum of the numbers for k d =1/2 (red) and k d =−1/2 (blue). ( b ) g 2 ( r ) for active (solid curve) and equilibrium (dashed curve) systems. Active system only exhibits algebraic order in low density regime. ( c , d ) Simulation snapshots for active system with ( c ) ρ =3.1 and ( d ) ρ =4.6. Note the transient excitation of vortex in d . ( e , f ) Driving-induced collision processes in highly dissipative system. The blue arrows indicate the direction of motion for particles on collision. Grey particles indicate the configurations before collision. Particle rotations depend on relative positions and angles between particles. In e , the colliding particle (red) tends to align with the collided particle (blue), while the collided particle tends to rotate away. In f , both particles align with each other. ( g , h ) Two different processes causing the instability of nematic alignment. Black lines indicate the bulk nematic alignment. Blue curves indicate the bending deformations of nematic alignment caused by fluctuations. Yellow arrows indicate the direction of motion for particles on collision. Green arrows indicate the direction of particle’s rotation caused by collision. Full size image As illustrated in Fig. 4e–h , we show the microscopic collision processes leading to order and dynamic instability in low and high density regimes, respectively. Figure 4e,f shows two basic modes of collision-induced rotations, which depend on relative positions and angles between particles [25] , [26] , [27] , [28] , [29] . Particles in Fig. 4e rotate in the same direction upon collision, which actually has no contribution to local alignment. The collision in Fig. 4f , however, causes a net alignment. This nematic alignment collision is extensively studied by simulation and kinetic theory [25] , [29] , [30] ; however, the effect of the collision process as shown in Fig. 4e on collective motion of active system is not well-understood. In Methods and Supplementary Discussion we give a detailed account of collision-induced rotations based on dynamic mean-field analysis. As given by Supplementary Equations (8) and (9) in Supplementary Discussion , the first terms on the right sides of these two equations give the rotations of the colliding (red) particles in Fig. 4e,f , whereas the second terms give the effect of rotations of the collided (blue) particles. Since the system is highly dissipative, the angular information exchanged upon collision holds long enough to facilitate order in low density, which causes enhanced ordering effect [26] . As shown in Supplementary Equation (23) in Supplementary Discussion , the isotropic nematic transition could take place at extremely low density if the rotational self-diffusion D r approaches zero. In simulations D r is set as 0, thus this analytical result explains the low density nematic order in simulations as shown in Fig. 4a . The calculations in Supplementary Discussion further reveal two typical ways causing dynamic instability in high-density regime. Supplementary Equation (28) in Supplementary Discussion shows that the linear instability of bending deformation leads to the breakdown of nematic order, and such instability has two contributions as illustrated in Supplementary Equations (18)–(20) in Supplementary Discussion . As shown in Fig. 4g , one process deforming nematic alignment is the rotation of particles triggered by collisions from two sides of the inflection region of bending fluctuations. Another process enhancing bending is shown at the peak or valley region of bending fluctuations in Fig. 4h . When particles in these region are colliding particles on their flanks, they tend to align with particles on each side, which further sharpens the local curvature. Abnormal density fluctuations and relaxations with defects The instability leads to the nonlinear spontaneous excitation of topological defect pairs. The separation of created topological defects induces large-scale bending and splay of nematic director field, which further drive large-scale particle flows [10] , [17] , [31] , [32] , [33] . The system is characterized by the nonperiodic recurrence of collective particle flows that span spatial-temporal scales much larger than that can be achieved by the individual constituent (see Supplementary Movie 2 ). Such state distinguishes from conventional steady state which requires constant fluxes. The collective swarming and swirling motions lead to highly dynamic density inhomogeneity and abnormal density fluctuations. To quantify the spatial property of such density inhomogeneity, we measure the root mean square deviation Δ N of a given area A by using the relation where g ( r ) is the radial distribution function and the integrals are performed over a region A with mean particle number (ref. 4 .) It is also measured directly by its definition (ref. 10 ). These two methods give the same results as shown in Fig. 5a , where Δ N / versus is plotted. In the regime <<1 (that is, Aρ 0 <<1), Δ N / varies as , since g ( r )=0 (for r < b , b is a particle’s semiminor axis) as a result of exclude volume effect. It explains why all the curves coincide and exhibit the first drop when <1 in Fig. 5a [34] , [35] . 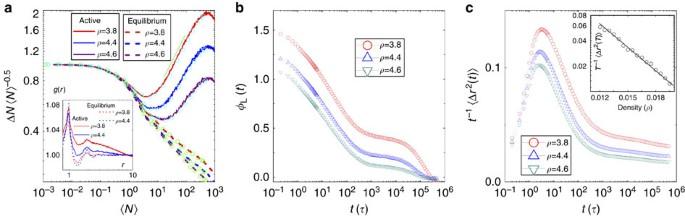Figure 5: Spatial and temporal characterization of giant number fluctuations. (a) Spatial number fluctuations are measured in active state (solid line) and compared with equilibrium simulations in the same densities (dashed line). Corresponding circles (cyan and green) show the results obtained by using Equation (1). (Inset) Typical radial distribution functiong(r) for active state (solid line) and equilibrium state (dashed line). (b) Multi-time scale relaxations of local number autocorrelations in active simulations. Logarithmic decays are observed in short-time regime. In the long-time regime the decay slows down and forms slowly declining floors. (c) Self-diffusion in active system. Super-diffusive, subdiffusive and normal diffusions are observed on different time regimes. (Inset) Density dependence of the long-time diffusive behaviour forT=4 × 105τ. Circles are simulation data and solid line indicates exponential decay. Figure 5: Spatial and temporal characterization of giant number fluctuations. ( a ) Spatial number fluctuations are measured in active state (solid line) and compared with equilibrium simulations in the same densities (dashed line). Corresponding circles (cyan and green) show the results obtained by using Equation (1). (Inset) Typical radial distribution function g ( r ) for active state (solid line) and equilibrium state (dashed line). ( b ) Multi-time scale relaxations of local number autocorrelations in active simulations. Logarithmic decays are observed in short-time regime. In the long-time regime the decay slows down and forms slowly declining floors. ( c ) Self-diffusion in active system. Super-diffusive, subdiffusive and normal diffusions are observed on different time regimes. (Inset) Density dependence of the long-time diffusive behaviour for T =4 × 10 5 τ . Circles are simulation data and solid line indicates exponential decay. Full size image Abnormal large fluctuations in active nematics are clearly illustrated when their curves diverge from the equilibrium cases for >1. Giant number fluctuations are observed for the case where quasi-long-range alignment becomes unstable. The green line in Fig. 5a , indicating Δ N , represents the most sharp increase of fluctuations we observe. With the increase of density, the system becomes more compact and the fluctuations decrease accordingly [34] . The giant number fluctuations found here is a result of the large-scale dynamic evolution of the strongly segregated patterns shown in Fig. 4d and Supplementary Movie 2 . Such evolution is driven by the deformation of nematic director fields as a consequence of the emergence of topological defects. The large voids found in Fig. 4d and Supplementary Movie 2 actually are just vortex defects or the combination of two +1/2 defects on the void’s boundary. To investigate the relaxation processes of abnormal fluctuations, we measure the autocorrelation , where n L ( t ) is the particle number in a given square of side length L at time t and is its average number. We also measure the particle’s time-dependent mean-square-displacement , which characterizes the dynamic property of particle motion. In short-time regime for t <200 τ, as shown in Fig. 5b , the autocorrelation ϕ L ( t ) shows fast logarithmic decay [10] . Correspondingly, as shown in Fig. 5c , in this regime first exhibits super-diffusive and consequent subdiffusive behaviour as a result of driving- and collision-induced local caged adjustments, respectively. In the long-time regime, the logarithmic decay of ϕ L ( t ) slows down after about 200 τ . This regime of slow decay coincides with the super-diffusive regime of topological defect k d =1/2 ( Fig. 1i ), and the height of the slowly declining floor is positively related to the strength of density inhomogeneity shown in Fig. 5a . They suggest a mutual correspondence between the relaxation of density inhomogeneities and the dynamics of topological defects. Furthermore, once topological defects are generated, they cannot be easily eliminated except through mutual annihilation. Such a conservative property make them play an important role in the large-scale collective dynamics of the system. After 10 5 τ , ϕ L ( t ) approaches zero and approaches the final diffusive behaviour, indicating that density inhomogeneities are not static and no stable constant global particle flows exist in the system, in accordance with seemingly random spontaneous behaviours of topological defects. Furthermore, the inset of Fig. 5c shows that the self-diffusivity decreases exponentially with the increase of particle density. This notable effect is also observed in experiments [36] . The following two aspects are of extreme importance for both the understanding and further application of active matter. The first is the emergence of new dynamic structures in active matter, which is impossible or difficult to realize in equilibrium. The second is the novel dynamics and functionality of specific structures in active matter. The study of active media thus is useful both for generating structures and realizing dynamical properties to fulfil novel functions unachievable in non-active media. In this study, we just focused on the above two aspects of topological defects in active nematics. Although topological defects may emerge both in active and non-active media, the dynamics of disclinations is qualitatively different in these two situations: polar disclination ( k d =1/2) in non-active nematics is found bound with disclination k d =−1/2, while in active nematics, it shows strong super-diffusive motion (see Fig. 1i ). In recent experiments of both driven granular rods and microtubules [7] , [10] , polar topological defects do show evidence of super-diffusive motions, although they are not critically determined by statistical measurement. On the other hand, the transportation behaviour of polar disclination in active nematics shows strong dynamical irreversibility that hinders the immediate annihilation of co-emerging polar and apolar disclinations. Local configuration of disclination pair determines the path to their annihilation or unbinding. Furthermore, the abnormal dynamics of topological defects not only drives the instability of quasi-long-range nematic order but also plays a critical role in the collective motion and giant number fluctuations in the system. After the spontaneous excitation, the polar disclination point will move away from the co-emerging apolar disclination. This process inevitably induces large-scale bending and splay of nematic director field, which further drive large-scale particle flows. Since the spontaneous excitation, active separation and annihilation of disclinations are genuinely aperiodic and endless, the system can only stay in a dynamical state with ever evolving large-scale particle flows. It distinguishes from conventional steady state which requires constant fluxes. The system is characterized by the non-periodic recurrence of collective particle flows that span spatial-temporal scales much larger than that can be achieved by its individual constituent. These collective swarming and swirling motions lead to highly dynamic density inhomogeneity and abnormal density fluctuations. More interestingly, by measuring the autocorrelation of local density and comparing with the corresponding spatial fluctuations, we reveal that the time regime for large-scale density relaxation coincides with the regime of super-diffusivity for polar disclinations. The density relaxation thus is organized by the motion of topological defects, which can be eliminated only by mutual annihilation. The dry system simulated here is different from active nematics in fluid media [37] , [38] , [39] , [40] . As a result of momentum conservation, in such wet active nematics, fluid flows driven by the activity of self-propelled particles play important roles in the collective motion of the system. Giomi et al. [39] recently show the drift motion of topological defects of k d =1/2 in extensile wet active nematics, and the so-called backflow is found playing an important role in defects dynamics. Alignment parameter (that is, flow aligning parameter [38] ) that serves as a feedback of fluid flow on nematic order is also found to be important for the emergence of topological defects [37] , [40] . The dry active nematics here, however, suggest a different mechanism for anomalous behaviour of topological defects. Collision-induced rotation is found important for the emergence of topological defects. Interestingly, we further identify weak polarity field near the topological defects, and its strength is found closely related to the drift speed of topological defects of k d =1/2. Such polarity field is enslaved to the spatial variation of nematic order and might play an important role in the evolution of topological defects, similar to the role of fluid flows in wet active nematics. In addition, the mean-field theory is used to helpfully understand the above nematic ordering and dynamic instability in low and high-density regimes, respectively. The present theory is similar to that of Baskaran and Marchetti on self-propelled rods [26] , [27] , [28] , and the major difference is that here a reversal rate of driving directions is applied. Furthermore, during the collision process, in their model they apply energy and momentum conserving law upon collision, but here we directly start from simple collision rules. In active system, due to the complexity of self-propelling entities and the frictions of substrate, the collision process does not conserve the kinetic energy and momentum. The present collision rules allow us to examine the effects of different collision processes on collective behaviours. There are two major collision processes in our theory. The nematic alignment collision process shown in Fig. 4f is widely used to explain the nematic ordering in driven rods system [25] , [29] , [30] , [32] . To our knowledge, the previous models that only include nematic alignment collision will not drive the active unbinding of topological defect pair as described here. On the other hand, our theory shows that the instability in the high-density regime is mainly caused by the collision process as shown in Fig. 4e . With such instability, the hydrodynamic theory of Ramaswamy et al. [17] on active nematics that predicts giant number fluctuations in 2D is not applicable in our situation. However, the observation of curvature driven flows still plays a critical role in large-scale relaxations. The major results of this paper can be readily tested in systems of driven granular rods and mobility assay experiments [6] , [7] , [8] , [10] . For further applications, our study suggests a way to control collective evolution in active media through tracking and manipulating topological defects in real time. For example, we could speed up or slow down the relaxation of density fluctuations by directly driving or pinning polar defects, respectively. It would be more interesting, if these could be achieved by adding particles of different dynamic properties. Such manipulations could be implemented both in future experiments and theoretical studies. Simulation In active simulation, the state of an ellipse particle j at simulation step n is denoted by the position of its centre of mass and the angle of major axis . We perform three basic trial operations on the position and angle of particles: where v 0 is the average velocity along the particle axis and . is +1 or −1, indicating that the particle is moving in the direction of or , respectively. will change or maintain its sign randomly every τ simulation sweeps on average through abiding by the Poisson distribution. is a delta-correlated vector white noise with its norm ≤1, and and are scalar white noises ( [0,1] and [−π/2,π/2]). In Equation (2), gives an average driving velocity v 0 . and together give a coloured noise with mean zero and a finite correlation time τ. Collision event takes place if the renewed space occupied by particle j overlaps with other particles. is 1 if particle j collides with or is collided by other particles during major-axial driving operation Equation (2) in step n −1, otherwise it is 0. Thus operations Equations (3) and (4) are collision-induced translational and rotational motions caused by major-axial driving. σ 1 and σ r are two parameters controlling the strengthes of translational and rotational motions, respectively. Taking hard-core interactions into consideration, the trial movements in Equations (2)–(4) are set to zero if the corresponding updated configurations overlap with other particles. Finally, the states of particles are updated as: In active simulations, the elliptic particles have the same aspect ratio as particles used in previously reported experiments [10] , that is, a / b =5.75, where a and b are semi major and minor axes of the particle, respectively. The major axis L =2 a is used as unit length. Periodic conditions are used in simulations with system size d =30. The dynamic parameters v 0 =0.012, σ 1 =0.004, σ r =0.015, and τ =6 are used in simulations unless otherwise indicated. We also perform classic equilibrium Monte-Carlo simulation using the same hard elliptic particles as those in active simulations. In equilibrium simulation, particles only perform translational and rotational movements conforming detailed balance to track physically most probable and realistic kinetic process. Defect identification and tracking To identify topological defects in simulations, we first assign an angle ϕ ( r ) on every site r of a square lattice. ϕ ( r ) is given through tanϕ( r )= , where w ( r − r i ) is a weight function and r i and θ i are the location and angle of the i th particle, respectively. In practice, we choose a gaussian form, w ( r − r i )= , where r ‖ and r ⊥ are the parallel and normal components of r − r i relative to the major axis of particle i [19] . Topological defects are identified by observing a net change of ϕ when we follow a closed loop on the lattice. The location of topological defects is determined by the centre of the smallest square with 2π (−2π) clockwise changes of ϕ. In analysis, the size of lattice is L /4, δ ‖ =2 a = L , and δ ⊥ =2 b . Dynamic mean-field theory To describe the spatial and angular number density distributions of particles, we introduce one-body distribution function f ± ( r , u , t ) for the particles that are driving in the direction of u or − u at time t , respectively. Further, we denote ω ± ( r , u , t ) as the collision-induced rotation rates of particles that are driving in the ± direction when the collision takes place. The most simplified dynamic mean-field equations that include the driving- and collision-induced rotation processes in the approximation of Itô-formalism [41] are given by where = u × ∂ u . The second term on the left-hand side of the equation represents the switching between two driving states with rate k ( 1/τ in simulation) and the third term is the instantaneous drift term with an average velocity v (= , where represents time average in simulation). On the right-hand side, the first term represents the self-rotational diffusion caused by driving noises, and the second term is the contribution of collision-induced rotations. Detailed analysis is given in Supplementary Fig. 1 and Supplementary Discussion . How to cite this article: Shi, X.-q. and Ma, Y.-q. Topological structure dynamics revealing collective evolution in active nematics. Nat. Commun. 4:3013 doi: 10.1038/ncomms4013 (2013).